Stable platinum nanoclusters on genomic DNA–graphene oxide with a high oxygen reduction reaction activity Nanosize platinum clusters with small diameters of 2–4 nm are known to be excellent catalysts for the oxygen reduction reaction. The inherent catalytic activity of smaller platinum clusters has not yet been reported due to a lack of preparation methods to control their size (<2 nm). Here we report the synthesis of platinum clusters (diameter ≤1.4 nm) deposited on genomic double-stranded DNA–graphene oxide composites, and their high-performance electrocatalysis of the oxygen reduction reaction. The electrochemical behaviour, characterized by oxygen reduction reaction onset potential, half-wave potential, specific activity, mass activity, accelerated durability test (10,000 cycles) and cyclic voltammetry stability (10,000 cycles) is attributed to the strong interaction between the nanosize platinum clusters and the DNA–graphene oxide composite, which induces modulation in the electronic structure of the platinum clusters. Furthermore, we show that the platinum cluster/DNA–graphene oxide composite possesses notable environmental durability and stability, vital for high-performance fuel cells and batteries. The oxygen reduction reaction (ORR) is attracting a great deal of attention in electrochemistry due to its technological importance in electrochemical energy conversion and storage devices, such as fuel cells [1] , [2] and secondary metal–air batteries [3] . Additionally, the ORR is important in water electrolysis, corrosion, diverse industrial processes and so on [4] , [5] , [6] . Conventionally, platinum (Pt) has been used as an active electrocatalyst for the ORR. However, the use of Pt in commercial applications as an electrocatalyst is limited due to scarce resources and high price [7] . Traditionally, electrochemical energy conversion and storage devices have suffered from poor ORR activity and stability. These factors make it necessary to develop a low-cost, highly active and durable electrocatalyst to improve the ORR performance. In this regard, the development of nanosize Pt clusters (Pt n ) as an electrocatalyst is highly demanded [8] , [9] . Synthesis and size control of nanosize Pt n is a great challenge, as such new methods for economically feasible large-scale production are still required [8] , [9] . As the activity of Pt catalysts in ORRs is influenced by the supporting material, an ideal supporting material should exhibit the following properties: high electrical conductivity; enhanced reactant gas contact with the electrocatalyst; adequate water handling capability at the cathode; good corrosion resistance; and high specific surface area. Graphene has attracted much interest in both fundamental and applied science since its 2004 discovery [10] and large-scale synthesis [11] , [12] , [13] . Owing to the sp 2 conjugation in the carbon lattice, electrons move ballistically in graphene even at ambient temperatures, showing excellent performance as electronic devices [14] , [15] . Graphene displays a high specific surface area (theoretical value, 2,620 m 2 g −1 ) [9] , good corrosion resistance and excellent conductivity [16] . The unique graphitic basal plane structure should guarantee its durability, as carbon materials with a large graphitic component are more durable [17] , [18] . Hence, graphene as a catalyst support would lead to an enhanced ORR catalytic activity and durability [19] . Keeping these important issues in mind, we have designed and synthesized a new highly durable Pt n /genomic double-stranded DNA–graphene oxide (Pt n /gDNA–GO)-based ORR electrocatalyst. We find that the Pt n /gDNA–GO composite maintains a high ORR onset potential, ORR half-wave potential, mass activity and specific activity, compared with that of Pt nanoparticles/GO and commercial state-of-the-art 20 wt% Pt/C (hereafter abbreviated as Pt/C; E-TEK, Somerset, NJ) catalysts. The Pt n /gDNA–GO composite exhibits excellent electrochemical stability compared with the Pt/C catalysts in acid medium. Additionally, the Pt n /gDNA–GO composite exhibits environmental stability and durability over a wide pH range. Synthesis The Pt n /gDNA–GO composites were prepared via a three-step synthesis as illustrated in Fig. 1 (see Methods for details). First, the gDNA–GO composites were prepared by mixing an aqueous dispersion of GO ( Supplementary Fig. S1a ) with a solution of gDNA ( Supplementary Fig. S1b ), followed by heating. During the heating process, the double-stranded DNA unwinds to form single-stranded DNA, which bridges adjacent GO nanosheets via strong noncovalent interactions. The gDNA–GO composite forms on cooling when the bases of the separate single-stranded DNA chains pair up with each other to reform the gDNA double-helix structure [20] . Second, Pt(terpy)Cl 2 [dichloro (2,2′:6′,2′′ terpyridine)platinum(II)] was added to the gDNA–GO suspension and incubated at 27 °C for 2 days. Studies have shown that the Pt(II) complexes can bind to the purine, guanine and adenine bases [21] , [22] . The two Cl − ions coordinated to the Pt 2+ ion are labile, therefore they are subsequently removed and the free coordination site available to the Pt 2+ ion coordinates with the purine bases and forms Pt 2+ –gDNA adducts. This coordination is well known to be due to the strong cation-π interaction between Pt 2+ and the purine ring [23] . Finally, the composite was reduced using NaBH 4 at 27 °C for 2 days, followed by dialysis. Reduction of Pt 2+ to Pt 0 led to the deposition of Pt n on GO as well as Pt nanoparticles in the gDNA, similar to metal reduction in electrochemically active calix nanotubes [24] , [25] . As a result, a very stable Pt n /gDNA–GO composite was formed via electrostatic interactions and deposition. 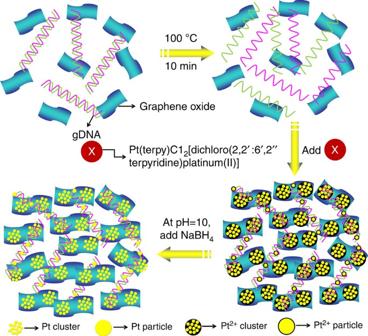Figure 1: Synthetic strategy. Schematic for preparing Ptn/gDNA–GO composites. Figure 1: Synthetic strategy. Schematic for preparing Pt n /gDNA–GO composites. Full size image Electrocatalyst characterization The synthesized products GO, gDNA–GO, Pt nanoparticles/GO and Pt n /gDNA–GO samples were characterized using Fourier transform infrared spectroscopy, X-ray photoelectron spectroscopy and energy dispersive X-ray ( Supplementary Methods ). The binding behaviour between gDNA and GO was analysed using Raman spectroscopy ( Supplementary Fig. S3 ). The peak positions at 1,350 and 1,600 cm –1 are ascribed to the D and G Raman bands of graphene, respectively ( Supplementary Fig. S3 ) [26] . In the case of gDNA–GO, the G Raman bands were observed at about 1,595 cm –1 . Owing to a small charge transfer from the nucleic acid bases of gDNA chains to GO, a red shift (~5 cm –1 ) is observed as compared with that of GO, this is similar to the case of wrapping carbon nanotubes with DNA [27] . The above result suggests that the gDNA is well-bound to the GO sheet. This correlates with the observed ultraviolet–visible results ( Supplementary Fig. S4 ). A red shift (~9 cm –1 ) is observed in the Pt nanoparticles/GO compared with that of gDNA–GO. This may be attributed to more significant charge transfer. Owing to a change in particle size, a blue shift (~6 cm –1 ) of the G band is observed for the Pt n /gDNA–GO composite as compared with that of Pt nanoparticles/GO [28] . This observed blue shift indicates that the Pt n firmly attaches to the surface of the gDNA–GO composite [29] . The attachment of the Pt particles and Pt n to the gDNA in the Pt n /gDNA–GO and Pt/gDNA catalysts is further confirmed by electrophoresis and energy-dispersive X-ray (EDX) analysis ( Supplementary Fig. S5a,b ). The structures of the GO, gDNA–GO, Pt nanoparticles/GO and Pt n /gDNA–GO samples were characterized using high-resolution scanning electron microscopy. In all of the samples, the continuous silk wave morphology associated with GO is observed due to strong interactions between the GO layers after evaporation of the solvent ( Supplementary Fig. S6 ) [30] , [31] . Owing to the small size of the Pt n and Pt nanoparticles, the Pt nanoparticles/GO and Pt n /gDNA–GO samples were analysed using low-resolution transmission electron microscopy (LRTEM) and high-resolution transmission electron microscopy (HRTEM). The LRTEM image of the surface of the Pt n /gDNA–GO composite shows Pt n evenly dispersed on the GO surface ( Supplementary Fig. S7a ). The HRTEM image of Pt n /gDNA–GO clearly shows well-defined single Pt n , as displayed in Fig. 2a . The sizes of indivisible Pt n are ~1 nm. Representative LRTEM and HRTEM images of the surface of the Pt nanoparticles/GO are shown in Fig. 2b and Supplementary Fig. S7b . The Pt nanoparticles are well dispersed with some agglomeration on the surface of GO. From HRTEM analysis, the size of individual nanoparticles are ~2–3 nm. In the case of Pt/C, the LRTEM image clearly shows an even dispersion of Pt nanoparticles on the surface of spherical carbon ( Supplementary Fig. S7c ). The HRTEM image ( Fig. 2c ) shows that the size of single nanoparticles are ~2–3 nm, similar to the Pt nanoparticles/GO sample. We further analysed nanocluster and nanoparticle size distributions from the HRTEM images of the Pt n /gDNA–GO composite, Pt nanoparticles/GO and Pt/C catalysts. A size distribution analysis of the Pt n reveals an average size of 1 nm, ranging from 0.8 to 1.4 nm ( Fig. 2d ). However, in the case of Pt nanoparticles/GO and Pt/C, the average size of the Pt nanoparticles is ~3 nm, ranging from 1 to 4–5 nm ( Fig. 2e,f ). 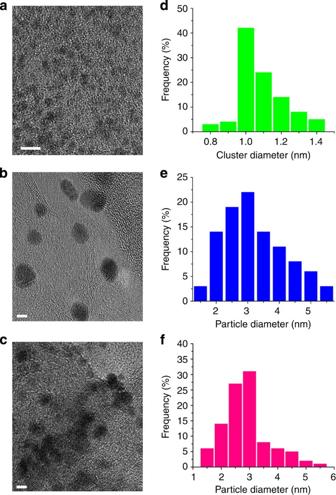Figure 2: TEM images and size histograms. (a–c) HRTEM images of the PtngDNA–GO composite, Pt nanoparticles/GO and Pt/C catalyst. Scale bars, 2 nm. (d) Histograms of Pt cluster sizes in the Ptn/gDNA–GO composite, (e) Pt particle sizes in the Pt nanoparticles/GO catalyst and (f) Pt particle sizes in the Pt/C catalyst. Figure 2: TEM images and size histograms. ( a – c ) HRTEM images of the Pt n gDNA–GO composite, Pt nanoparticles/GO and Pt/C catalyst. Scale bars, 2 nm. ( d ) Histograms of Pt cluster sizes in the Pt n /gDNA–GO composite, ( e ) Pt particle sizes in the Pt nanoparticles/GO catalyst and ( f ) Pt particle sizes in the Pt/C catalyst. Full size image Electrocatalytic performance The catalytic activity of the Pt n /gDNA–GO composite was compared with the Pt nanoparticles/GO and Pt/C catalysts. Cyclic voltammetry (CV) curves for the catalysts at room temperature in N 2 -saturated 0.1 M HClO 4 are shown in Supplementary Fig. S14 . The CV curves exhibit two distinctive potential regions associated with the under-potentially deposited hydrogen (H upd ) adsorption/desorption processes (H + +e – =H upd ) between 0< E <0.37 V and the formation of an OH ad layer (2H 2 O=OH ad +H 3 O + +e – ) beyond ~0.6 V (ref. 32 ). The specific electrochemically active surface area (EASA) was calculated by measuring the charge collected in the H upd adsorption/desorption region after double-layer correction, and assuming that a constant 0.21 mC cm −2 charge is required to oxidize a monolayer of H 2 on a polycrystalline Pt electrode (see Supplementary Methods ). The specific EASA of theses catalysts were measured to be 66.6, 57.3 and 74.1 m 2 g −1 for the Pt n /gDNA–GO composite, Pt nanoparticles/GO and Pt/C catalyst, respectively. We further performed CO-stripping CV ( Supplementary Methods ) to obtain the accurate catalytic activity. Representative CO-stripping CV curves for the Pt n /gDNA–GO, Pt nanoparticles/GO and Pt/C catalysts are shown in Supplementary Fig. S15 . The calculated EASA area of Pt nanoparticles/GO and Pt/C are ~59.1 and ~73.4 m 2 g −1 , respectively. This value is calculated by integrating the CO oxidation peak of the first CO-stripping cycle, assuming an oxidation charge value of 420 μC cm −2 for a monolayer of CO adsorbed on a smooth Pt surface [33] , [34] , [35] , [36] , [37] , [38] . However, the EASA area of Pt n /gDNA–GO is ~149.8 m 2 g −1 , which is more than double that estimated from the H upd adsorption/desorption experiments. This discrepancy in the EASA values determined from H upd adsorption/desorption and from CO-stripping experiments could be due to the presence of a large double-layer charge in GO. This increased ESA of the Pt n /gDNA–GO can significantly improve catalytic activity towards the ORR compared with the other two catalysts. The ORR catalytic activity and kinetics in an O 2 -saturated 0.1 M HClO 4 solution were studied by using a glassy carbon rotating-disk electrode at room temperature. Polarization curves for the ORR on these three catalysts are displayed in Fig. 3a–d and Supplementary Fig. S16a–d . The onset potentials for the ORR are ~1.01, ~0.99 and ~0.95 V for the Pt n /gDNA–GO composite, Pt nanoparticles/GO and Pt/C, respectively. A higher ORR half-wave potential was observed for the Pt n /gDNA–GO composite (~0.90 V) compared with the Pt nanoparticles/GO (~0.83 V) and Pt/C (~0.85 V) catalysts. The increased onset and half-wave potential observed in the Pt n /gDNA–GO composites are due to the reduction of O 2 molecules via Pt n as well as the Pt nanoparticles fixed in the purine bases ( Supplementary Fig. S17 ). Pt nanoparticles/GO shows a lower current density of 0.9 V ( Supplementary Fig. S16a ) than the Pt n /gDNA–GO composite. This indicates that the kinetic current is lower when Pt nanoparticles are loaded on GO. Additionally, the diffusion-limiting potential region is short for the Pt nanoparticles/GO, resulting in a faster kinetic current drop with increasing potential. For the Pt n /gDNA–GO composite ( Fig. 3a ), the mixed kinetic-diffusion control region occurs between 0.75 and 1.01 V, which is higher than that of the Pt/C catalyst (between 0.7 and 0.9 V, Supplementary Fig. S16b ). As represented in Fig. 3c , the Pt n /gDNA–GO composite showed a mass activity of 0.317 mA μg metal −1 at 0.9 V versus a reversible hydrogen electrode. This value is 3.3 and 2.6 times higher than that of the Pt/C (0.096 mA μg metal −1 , Fig. 3c ) and the Pt nanoparticles/GO (0.121 mA μg metal −1 , Fig. 3c ) catalyst, respectively. Our Pt n /gDNA–GO composite displays one of the highest mass activities for the ORR ( Supplementary Table S3 ). 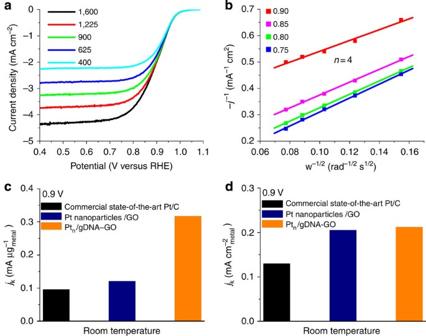Figure 3: ORR catalytic properties. (a) ORR polarization curves of the Ptn/gDNA–GO composite in an O2-saturated 0.1 M HClO4solution with a sweep rate of 10 mV s−1at different rotation speeds. (b) Corresponding K–L plots at different potentials. (c) Mass activity and (d) specific activity at 0.9 V versus reversible hydrogen electrode (RHE) for different catalysts. Mass and specific activities are given as kinetic current densities (jk) normalized in reference to the loading amount of metal and EASA (EASA from CO stripping), respectively. The metal loading on the rotating-disk electrode was ~11.3 μg cm−2for Ptn/gDNA–GO, Pt nanoparticles/GO and Pt/C. Inathe current density was normalized in reference to the geometric area of a rotating-disk electrode (0.0707, cm2). Figure 3: ORR catalytic properties. ( a ) ORR polarization curves of the Pt n /gDNA–GO composite in an O 2 -saturated 0.1 M HClO 4 solution with a sweep rate of 10 mV s −1 at different rotation speeds. ( b ) Corresponding K–L plots at different potentials. ( c ) Mass activity and ( d ) specific activity at 0.9 V versus reversible hydrogen electrode (RHE) for different catalysts. Mass and specific activities are given as kinetic current densities ( j k ) normalized in reference to the loading amount of metal and EASA (EASA from CO stripping), respectively. The metal loading on the rotating-disk electrode was ~11.3 μg cm −2 for Pt n /gDNA–GO, Pt nanoparticles/GO and Pt/C. In a the current density was normalized in reference to the geometric area of a rotating-disk electrode (0.0707, cm 2 ). Full size image The Pt n /gDNA–GO composite had a specific activity (that is, kinetic current per unit surface area of catalyst) of 1.63 times that of the Pt/C catalysts and 1.03 times that of the Pt nanoparticles/GO ( Fig. 3d ). Linearity in Koutecky–Levich (K–L) plots, as well as parallelism of the fitting lines is known to correspond to first-order reaction kinetics with respect to concentration of dissolved O 2 molecules [39] . From the slopes of the K–L plots ( Fig. 3b ), the number of electrons transferred ( n ) during the ORR was calculated to be ~4.0 at 0.75–0.9 V for the Pt n /gDNA–GO composite, which is similar to the number of electrons transferred using the Pt/C catalyst ( n ~3.7, Supplementary Fig. S16d ). The increased ORR onset potential, half-wave potential, mass activity and specific activity exhibited by the Pt n /gDNA–GO composite could be due to significant changes in the active surface area of Pt n and chemical interactions between Pt and GO, which can alter the electron density in the d -orbitals of Pt, thereby enhancing the ORR catalytic activity. Additionally, a more facile transport of the reduced species occurs in the gDNA–GO composites, due to strong binding between gDNA and GO, which creates an increased electronic conductivity and corrosion resistance. Accelerated degradation tests (ADTs) were conducted by cycling the catalysts in an O 2 -saturated HClO 4 solution at 0.6 and 1.2 V at a sweep rate of 50 mV s −1 , while CV curves between 0 and 1.4 V were recorded to compare the EASA during potential cycling. 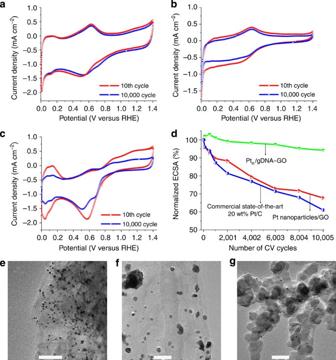Figure 4: ADT and TEM microstructure of the catalysts after ADT. CV curves of 10th and 10,000 cycle for the (a) Ptn/gDNA–GO composite, (b) Pt nanoparticles/GO and (c) Pt/C catalyst. (d) Comparison of decrease in EASA for the catalysts. The durability test was carried out for the three samples in an O2-saturated 0.1 M HClO4solution with the cyclic potential sweeping between 0.6 and 1.2 V versus reversible hydrogen electrode (RHE) at a scan rate of 50 mV s−1. The metal loading on the rotating-disk electrode was 11.3 μg cm−2and current densities were normalized in reference to the geometric surface area of a rotating-disk electrode (0.0707, cm2). (e–g) TEM images of the Ptn/gDNA–GO, Pt nanoparticles/GO and Pt/C catalyst after the ADT. Scale bars, 20 nm. Figure 4a–c show the 10th and 10,000 CV curves for the Pt n /gDNA–GO composite, Pt nanoparticles/GO and Pt/C catalysts. After cycling, the CV measurements showed a loss of ~5.8% in EASA for the Pt n /gDNA–GO composite, ~39% for the Pt/C and ~33% for the Pt nanoparticles/GO catalyst ( Fig. 4d ). ORR activities after the ADT were measured for all samples in O 2 -saturated HClO 4 solution. Supplementary Fig. S18a–c show the polarization curves for the Pt n /gDNA–GO composite, Pt nanoparticles/GO and Pt/C catalyst before and after the ADT. In the mixed kinetic-diffusion control region, the Pt nanoparticles/GO and Pt/C catalyst show a large current drop after the ADT, while there is almost no change for the Pt n /gDNA–GO composite ( Supplementary Fig. S18a–c ). To reveal the mechanism of the durability enhancement, the catalysts were collected by sonicating the glassy carbon disk electrode in ethanol after the ADT, and their structures were observed by transmission electron microscopy (TEM; Fig. 4e–g ). The Pt nanoparticles/GO catalyst shows an increase in nanoparticle size from ~3 to ~20 nm after the ADT ( Fig. 4f ), while the Pt/C catalyst shows an increase in size from ~3 to ~10 nm after the ADT ( Fig. 4g ). The increase in Pt nanoparticle size is due to Ostwald ripening, which is consistent with the observed decrease in EASA for these catalysts. Additionally, fewer nanoparticles are observed in the Pt nanoparticles/GO and Pt/C samples after the ADT test. This is due to corrosion of GO and carbon, which leads to the detachment of Pt nanoparticles from the support material. In contrast, the Pt n /gDNA–GO composite displayed the same features before and after the ADT ( Supplementary Fig. S18a ) with Pt n sizes between 1.0 and 1.5 nm and uniform nanoparticle distribution ( Fig. 4e ). Figure 4: ADT and TEM microstructure of the catalysts after ADT. CV curves of 10th and 10,000 cycle for the ( a ) Pt n /gDNA–GO composite, ( b ) Pt nanoparticles/GO and ( c ) Pt/C catalyst. ( d ) Comparison of decrease in EASA for the catalysts. The durability test was carried out for the three samples in an O 2 -saturated 0.1 M HClO 4 solution with the cyclic potential sweeping between 0.6 and 1.2 V versus reversible hydrogen electrode (RHE) at a scan rate of 50 mV s −1 . The metal loading on the rotating-disk electrode was 11.3 μg cm −2 and current densities were normalized in reference to the geometric surface area of a rotating-disk electrode (0.0707, cm 2 ). ( e – g ) TEM images of the Pt n /gDNA–GO, Pt nanoparticles/GO and Pt/C catalyst after the ADT. Scale bars, 20 nm. Full size image The long-term stabilities of the catalysts were determined by CV cycling in a N 2 -saturated 0.1 M HClO 4 solution between 0 and 1.4 V. Supplementary Fig. S19a–c shows the 20th and 10,000 CV curves for the catalysts, and a clear decrease in activity is observed for the Pt nanoparticles/GO and Pt/C catalysts. For a clear observation of CV stability, the normalized EASA for the catalysts was plotted (versus 20 cycles) as a function of the number of CV cycles ( Supplementary Fig. S19d ). A decrease in EASA of ~6%, compared with the initial EASA, is observed for Pt n /gDNA–GO composite after 10,000 cycles, while a decrease in EASA of ~48% and ~60% is observed for the Pt nanoparticles/GO and Pt/C catalysts, respectively. The results of the long-term stability test are consistent with the findings of the ADT test. The observed enhanced stability can be due to the strong interaction between Pt n , gDNA and GO. The Pt n are stabilized by coordination with the purine moieties in the gDNA as well as graphene [40] , [41] . Environmental and pH stability The long-time environmental stability of the Pt n /gDNA–GO composite at various pH conditions (pH=1–13) was conducted ( Fig. 5a ). It can be seen that the Pt n /gDNA–GO composite is stable under these harsh environmental conditions at room temperature for 2 months. Besides the visually observed environmental stability, we also performed ORR activity experiments over a wide range of pH values ( Fig. 5b ). As can be seen in Fig. 5b , the Pt n /gDNA–GO composite displayed a constant relative mass activity over a wide pH range (1–13 pH), which means that the composite is extremely stable at various pH values. On the other hand, the ORR relative mass activities for Pt nanoparticles/GO and Pt/C catalysts ( Fig. 5b ) vary as the pH changes, which is likely to arise from the instability of the composites at various pH values. This excellent environmental and pH stability of the Pt n /gDNA–GO composite could be attributed to the strong binding of the gDNA chains to GO sheets through multiple noncovalent interactions. These noncovalent interactions include π−π stacking [42] between the bases of gDNA and graphitic domains of GO sheets, as well as hydrogen bonding between the amines of the gDNA bases and the oxygen-containing functional groups of the GO sheets [43] . 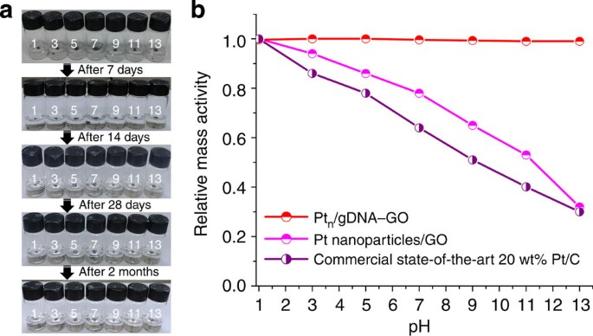Figure 5: Solution phase and pH stability. (a) Effects of pH on the Ptn/gDNA–GO composite. The pH value is numbered on each bottle. The Ptn/gDNA–GO composite was placed into the respective solutions, and allowed to stand at room temperature for 8 weeks. (b) The relative mass activity of the catalysts measured in O2-saturated electrolytes of varying pH with a scan rate of 10 mV s−1at a rotation speed of 1,600 r.p.m. Figure 5: Solution phase and pH stability. ( a ) Effects of pH on the Pt n /gDNA–GO composite. The pH value is numbered on each bottle. The Pt n /gDNA–GO composite was placed into the respective solutions, and allowed to stand at room temperature for 8 weeks. ( b ) The relative mass activity of the catalysts measured in O 2 -saturated electrolytes of varying pH with a scan rate of 10 mV s −1 at a rotation speed of 1,600 r.p.m. Full size image Herein we described the synthetic method to produce a novel Pt n /gDNA–GO composite. The synthesized composite was characterized by Fourier transform infrared (FTIR), Raman, ultraviolet–visible, scanning electron microscopy, TEM, HRTEM, EDX and X-ray photoemission spectroscopy (XPS), which clearly demonstrate that the Pt n /gDNA–GO composite is successfully synthesized. The interactions between gDNA and GO may provide an efficient approach for positioning Pt ions to form the Pt nanoclusters on the surface of GO. Thus, gDNA holds great promise as a cost-effective and environmentally friendly template for large-scale production of Pt n /GO. This newly developed method suggests a technique to synthesize other types of GO-supported nanoclusters, such as Ag, Pd, Au and so on. The electrochemical data show that the as-synthesized Pt n /gDNA–GO composite exhibits a greater ORR onset potential, ORR half-wave potential, specific activity and mass activity for the ORR compared with Pt nanoparticles/GO and Pt/C catalysts. The Pt n /gDNA–GO composite displays an excellent accelerated durability test (10,000 cycles) and a long-term CV stability (10,000 cycles) as compared with Pt nanoparticles/GO and Pt/C catalysts in acidic media. Furthermore, good corrosion resistance and high conductivity of Pt n /gDNA–GO composites may account for the observed enhanced performance. These properties make us believe that the Pt n /gDNA–GO composites might have a promising future in applications such as fuel cells, supercapacitors, biosensors, nanoscale electronics, drug delivery and imaging of cancer cells [44] , [45] , [46] , [47] . This is due to their ability to promote faster oxygen reduction kinetics, their robustness against environmental degradation and electrochemical stability. Genomic double-stranded deoxyribonucleic acid Application of pure gDNA in material sciences has added a new horizon to the conventional materials science landscape. To obtain pure gDNA from plant leaves at a large scale is likely to be a difficult task due to accumulation of polysaccharide and phenolic compounds. In this regard, we took advantage of the model plant Arabidopsis thaliana , which contains a smaller amount of polysaccharide and phenolic compounds, to isolate gDNA on a large scale. The A 260 /A 280 ratio of gDNA was 1.83, which shows that the large-scale isolated gDNA (6 mg ml −1 ) was pure enough to use in the present study. Isolated gDNA was subjected to hydrodynamic shearing by exposure to brief periods of sonication to generate gDNA fragments of size 300–700 base pairs (bp; Supplementary Fig. S1d ). Utilizing a specific sonication cycle we successfully sheared more than 95% of the total gDNA to the expected size ( Supplementary Fig. S1d : lanes 1 and 2, and lane 3 lower bands) compared with unsonicated gDNA ( Supplementary Fig. S1d : lane 3 upper band). The detailed procedures for isolation of gDNA and synthesis of GO are given in Supplementary information . Synthesis of gDNA–GO composites To an aqueous GO (200 mg/50 ml) dispersion, 4 ml of an aqueous gDNA solution (6 mg ml −1 ) was added and the mixture was sonicated for 4 h. Finally, the mixture was heated at 100 °C for 10 min. After cooling to room temperature, the gDNA–GO composite solution was kept for further reactions. Synthesis of Pt n /gDNA–GO composites and Pt nanoparticles/GO The synthesis of 20 wt% Pt n /gDNA–GO composites involved mixing 110 mg of Pt(terpy)Cl 2 [dichloro(2,2′:6′,2′′ terpyridine)platinum(II)] with 54 ml of a gDNA–GO suspension followed by incubation at 27 °C for 2 days with vigorous stirring. Finally, 50 ml NaBH 4 aqueous solution with a concentration of 5 mg ml −1 was added and reduction was allowed to proceed for 2 days at 27 °C. At the end of the experiments, the solution was dialysed through cellulose membranes to remove free Pt and NaBH 4 ions that were not bound to the gDNA–GO composites. For the synthesis of 20 wt% Pt nanoparticles/GO the same procedure was followed, with a gDNA–GO suspension replaced by a GO suspension. The schematic diagram for the synthesis of Pt nanoparticles/GO composites is depicted in Supplementary Fig. S20 . Characterization Atomic force microscopy (AFM) images were recorded using an AFM, Bruker-N8 NEOS. The sample was prepared by depositing an aqueous GO dispersion onto a clean silicon surface and then drying the sample under vacuum at room temperature. The gDNA AFM sample was prepared by dropping a 1.0 ml of extracted gDNA solution directly onto to a clean silicon surface. FTIR spectra were recorded in KBr pellets using a Bruker FTIR. Measurements of micro Raman spectra were carried out using a Senterra Raman Scope system with a 532-nm wavelength incident laser light and 20 mW power. Ultraviolet–visible absorption spectra were recorded with a Shimadzu UV–2401PC spectrophotometer. The samples were dispersed in deionized (DI) water for optical measurements. The morphologies of the resulting products were characterized using a field-emission scanning electron microscope (JEOL, FEG–XL 30S) with an acceleration voltage of 5 KV. LRTEM and HRTEM observations were carried out in a JEM-2200FS (Cs corrected STEM) electron microscope with an accelerating voltage of 200 kV. The TEM specimens were prepared by dispersing the platinum clusters/particles on a copper grid. XPS analysis was performed with an ESCALAB–220I–XL (Thermo–Electron, VG Company) device. XPS was used to characterize the GO, gDNA–GO, Pt nanoparticles/GO, Pt/C and Pt n /gDNA–GO catalysts after deposition of the as-synthesized samples onto a silicon wafer. Electrochemical characterization CVs were recorded by scanning the electrode potential from 0.0 to 1.4 V (versus reversible hydrogen electrode) at a scan rate of 50 mV s −1 . The VSP-Modular 2 Channels Potentiostat/Galvanostat/EIS (Bio-Logic Science Instruments) was calibrated with respect to an Ag/AgCl electrode. CV measurements were carried out in an N 2 -saturated 0.1 M HClO 4 solution at room temperature. Rotating-disk electrode measurements were carried out in an O 2 -saturated 0.1 M HClO 4 solution at room temperature using a rotating-disk electrode system for ORR calibration. Linear sweep voltammograms were recorded by scanning the disk potential from 1.1 to 0.4 V (versus reversible hydrogen electrode) at a scan rate of 10 mV s −1 . For CV and rotating-disk electrode experiments, a three-electrode configuration was used, consisting of a modified glassy carbon electrode (geometric area of 0.0707, cm 2 ) as the working electrode, Ag/AgCl electrode and Pt wire as a counter electrode. See Supplementary Methods for further details. How to cite this article: Tiwari, J. N. et al . Stable platinum nanoclusters on genomic DNA–graphene oxide with a high oxygen reduction reaction activity. Nat. Commun. 4:2221 doi: 10.1038/ncomms3221 (2013).